Si:P as a laboratory analogue for hydrogen on high magnetic field white dwarf stars Laboratory spectroscopy of atomic hydrogen in a magnetic flux density of 10 5 T (1 gigagauss), the maximum observed on high-field magnetic white dwarfs, is impossible because practically available fields are about a thousand times less. In this regime, the cyclotron and binding energies become equal. Here we demonstrate Lyman series spectra for phosphorus impurities in silicon up to the equivalent field, which is scaled to 32.8 T by the effective mass and dielectric constant. The spectra reproduce the high-field theory for free hydrogen, with quadratic Zeeman splitting and strong mixing of spherical harmonics. They show the way for experiments on He and H 2 analogues, and for investigation of He 2 , a bound molecule predicted under extreme field conditions. The response of atoms to high magnetic fields has been of interest for many decades [1] , [2] , [3] , [4] . It has been suggested that magnetic flux densities up to 10 5 T (1 gigagauss) exist on the surface of white dwarf and cataclysmic variable stars [5] , [6] , [7] . This inference is based on a complex process that involves a combination of modelling the pattern of flux around the surface and up through the atmosphere of the star, and a search for transitions that are stationary with magnetic field [2] , [3] , [4] . These models are then compared with astrophysical spectra. Definitively extracting a magnetic field value from the comparison is challenging because the measured spectra are noisy with many overlapping features, as can be seen from some examples in Fig. 1 . In some cases, predicted features are missing and in others there are extra features. Such discrepancies are usually attributed to the inhomogeneity of the magnetic field across the surface or line-of-sight, and possibly species other than hydrogen. At the same time, there is controversy about how such high fields could even persist for any significant length of time [8] , and the dearth of high-field magnetic white dwarfs (HFMWDs) found in binary systems [9] . Identification of the observed spectral features is further hindered at these fields because the calculation of theoretical spectra where the magnetic cyclotron energy ( ħeB / m e ) is comparable to the coulombic binding energy (the Rydberg R = m e e 4 /2 κ 2 ħ 2 , where κ =4 πɛ 0 ) is non-trivial, especially for atomic species other than hydrogen, such as helium [10] , [11] , [12] . The difficulty is that in the regime of interest ( B ~ B 0 = m e 2 e 3 /2 κ 2 ħ 3 ) the Zeeman effect becomes quadratic [13] , [14] , [15] , the spherical symmetry of the Coulomb potential competes with the cylindrical symmetry of the magnetic field, and the Schrodinger equation is non-integrable, so producing quantum chaos [16] , [17] . The theory for the very complex Zeeman structure in atoms has been compared with laboratory absorption spectra in magnetic fields up to 8 T (refs 13 , 14 , 15 ). Although in Rydberg atoms the cyclotron energy can be more easily made equivalent to the substantially lower binding energy (the characteristic field is lowered by a factor n 4 where n is the principal quantum number) [18] , the regime near B 0 is receiving renewed interest because it has recently been shown that a new kind of magnetic chemical bond can be produced that supersedes the electronic bond [19] , creating new molecules such as He 2 . 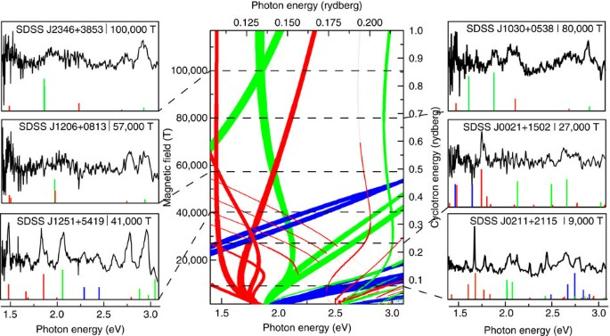Figure 1: Hydrogen Balmer spectrum for HFMWDs. The spectra are taken from the Sloane Digital Sky Survey7. They have been flattened by subtracting a 4th order polynomial fit and inverted. Also shown are all theoretical Balmer series transitions—we have chosen the field values to produce the best fit. No account has been taken here of the temperature or the spatial and temporal field inhomogeneity and this accounts for the difference in the field values quoted here when compared with fits from a full calculation7. The magnitude of the dipole matrix element, and the polarization are shown, respectively, by the length and colour of the lines (red, circularσ+polarization, Δm=−1; green, linearπz, Δm=0; blue, circularσ−, Δm=+1). Figure 1: Hydrogen Balmer spectrum for HFMWDs. The spectra are taken from the Sloane Digital Sky Survey [7] . They have been flattened by subtracting a 4th order polynomial fit and inverted. Also shown are all theoretical Balmer series transitions—we have chosen the field values to produce the best fit. No account has been taken here of the temperature or the spatial and temporal field inhomogeneity and this accounts for the difference in the field values quoted here when compared with fits from a full calculation [7] . The magnitude of the dipole matrix element, and the polarization are shown, respectively, by the length and colour of the lines (red, circular σ + polarization, Δ m =−1; green, linear π z , Δ m =0; blue, circular σ − , Δ m =+1). Full size image The Hamiltonian for an electron in atomic hydrogen usually applied is where p =− iħ is the momentum operator. When a hydrogen atom is subjected to a magnetic field, we replace p 2 in equation 1 by ( p + A ) 2 , where A is the vector potential defined by B = × A . We now have, in units such that m e = e=κ=ħ= 1, where H 0 is the zero-field Hamiltonian (equation 1), the second term, H 1 , is linear in field and the last term, H 2 , is responsible for the quadratic Zeeman effect. The Hamiltonian of equations 1 and 2 ignores spin orbit coupling and assumes the heavy ion mass limit, that is, it ignores the motion of the ion/donor. The general case is considered in refs 20 , 21 . In other species, different approximations are necessary. Given the above questions, and the renewed interest in the high-field regime, it is crucial to validate experimentally the theory for the absorption spectra on which the inferred fields are based. Doing so directly for hydrogen is impractical because the required fields are two to three orders of magnitude beyond what is currently available in any laboratory [22] , [23] . Such tests become even more essential where atomic species beyond hydrogen are being considered, for example, helium [10] , [11] , [12] or molecular hydrogen [24] , [25] , [26] , [27] as for these cases the multiple particle calculations required are complex and involve approximations (for example, basis-state choices and sizes) that are not a priori guaranteed. In low field, the Zeeman spectrum may be found from perturbation theory, the orbital and magnetic quantum numbers are constants of the motion. In this regime, B«B 0 (half an atomic unit of field) the quadratic term is negligible, and the transitions shift linearly with field because H 1 =½ L z B z produces the usual linear Zeeman energy ½ mB (where L z is the component of angular momentum along B || z and m is the magnetic quantum number). At very high field, the Coulomb potential is the perturbation and again there are constants of motion, but in the intermediate regime close to B 0 , the Zeeman spectrum is much more complex ( Fig. 1 ). It has long been known [1] that shallow impurities in semiconductors exhibit energy level spectra that bear striking similarities to those of free atoms, and the canonical example is the Group V donor such as phosphorus in silicon (Si:P). In this case, the Group IV silicon atoms are tetrahedrally bonded, so the donor has one unused valence electron, loosely bound, which orbits about the ion core. The Si:P system yields well-resolved hydrogenic Lyman series spectra at zero field [28] , [29] with excitations that are long lived and useful as alternatives to free atoms for quantum information applications [30] , [31] , [32] . The cyclotron energy and the donor-binding energy are equal for magnetic fields at around 30 T because the cyclotron and binding energies are scaled by the effective mass and dielectric constant [1] , [33] . Equation 2 still holds, and we now use appropriately scaled units so that m*=e=ɛ r κ=ħ= 1, see Table 1 . Table 1 Experimental parameters and derived units. Full size table There are other possible analogues such as acceptors but these are much more complicated [34] , while other host materials such as III–V semiconductors generally produce such a small binding energy, or such wide homogeneous line widths, that the Rydberg states are not well resolved until B»B 0 (refs 33 , 35 ), which thus sheds little light on the understanding of HFMWDs. To validate any computational scheme for helium in the high magnetic field regime accurately, a suitable analogue to measure would be the double donor sulphur in Si (ref. 36 ). Similarly, the ability to position phosphorous donors with atomic precision allows one to build coupled donor pairs to mimic molecular hydrogen [24] , [25] , [26] , [27] . In this work, we use Si:P as an analogue of hydrogen in conditions similar to those at the surface of HFMWDs. The measured Lyman series spectra reproduce the theoretical predictions for free hydrogen under high field, with quadratic Zeeman splitting and strong mixing of spherical harmonics, demonstrating the possibility of the use of Si:P for modelling astrophysical data in the laboratory. 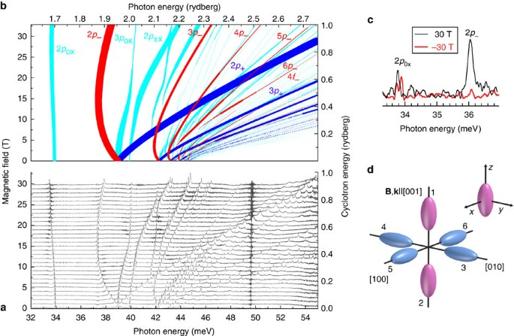Figure 2: Field dependence of Si:P Lyman series. The field was oriented along the [001] crystal axis in Faraday geometry (that is, light propagation along the field axis). The sample temperature was 2.2 K (so thatkBT=0.010 Rydberg, equivalent to 1,600 K for free hydrogen atoms). (a) Experimental far-infrared absorption spectra. Each transmission spectrum has been normalized, then inverted and finally offset so that the baseline corresponds to the field applied. No smoothing or other processing has been used. The noise feature just below 50 meV that increases in size with field is due to vibrations in the magnet cooling water system. (b) Theoretical donor Lyman transition spectrum. The strongest transitions are labelled according to their upper state. The magnitude of the dipole matrix element and polarization are indicated, respectively, by the thickness and colour of the lines (red, circularσ+for valleys 1 and 2; blue, circularσ–for valleys 1 and 2; cyan, unpolarized transitions for valleys 3–6). Some important states have been identified from the dominant components of the wavefunction character. Note that the 4f–state labelled at about 20 T is only weakly allowed and undergoes many anti-crossings with thep–series. (c) Circularly polarized absorption spectrum. (d) The multi-valley conduction band of silicon. The valley axis coordinate system (x,y,z) and the light propagation (k) and field (B) directions used are indicated. High-field Lyman spectroscopy of Si:P Figure 2 shows the measured and computed Lyman series spectra for silicon doped with phosphorus as a function of applied magnetic field (see Supplementary Data 1 for the raw data). The [001] cubic crystal axis, the field and the light propagation direction were chosen to be all parallel (Faraday geometry). The circular polarization dependence of the lowest two transitions is also shown in Fig. 2 , for forward and reverse fields ( Supplementary Data 2 ), showing that some transitions select one circular polarization. The experimental donor transitions are sharp and clearly resolved up to principal quantum number n =6. Figure 2: Field dependence of Si:P Lyman series. The field was oriented along the [001] crystal axis in Faraday geometry (that is, light propagation along the field axis). The sample temperature was 2.2 K (so that k B T =0.010 Rydberg, equivalent to 1,600 K for free hydrogen atoms). ( a ) Experimental far-infrared absorption spectra. Each transmission spectrum has been normalized, then inverted and finally offset so that the baseline corresponds to the field applied. No smoothing or other processing has been used. The noise feature just below 50 meV that increases in size with field is due to vibrations in the magnet cooling water system. ( b ) Theoretical donor Lyman transition spectrum. The strongest transitions are labelled according to their upper state. The magnitude of the dipole matrix element and polarization are indicated, respectively, by the thickness and colour of the lines (red, circular σ + for valleys 1 and 2; blue, circular σ – for valleys 1 and 2; cyan, unpolarized transitions for valleys 3–6). Some important states have been identified from the dominant components of the wavefunction character. Note that the 4 f – state labelled at about 20 T is only weakly allowed and undergoes many anti-crossings with the p – series. ( c ) Circularly polarized absorption spectrum. ( d ) The multi-valley conduction band of silicon. The valley axis coordinate system ( x,y,z ) and the light propagation ( k ) and field ( B ) directions used are indicated. Full size image Theoretical field dependence of Si:P and free hydrogen Figure 1 shows the positions and dipole transition strengths of the Balmer series for known HFMWDs, and Fig. 3 the Lyman series. Whereas the low field limit of the Balmer series has only three components that split linearly, at high field, the Hα (2 p- 3 d ) line splits into 3 × 5=15 components and so on. The quadratic Zeeman effect produces transitions that are forbidden at low field and a very complex Balmer spectrum ( Fig. 1 ). The complexity is only somewhat reduced in the Lyman series ( Fig. 3 ). Figure 2 shows the theoretical field dependence of the Si:P transition energies. The absolute level positions were calculated in atomic units, and these were converted to transition energies using a field-independent ground state energy of −2.277 R (see below). The magnetic field and transition energies were converted to tesla and meV using standard parameters ( Table 1 ), so no fitting was performed. 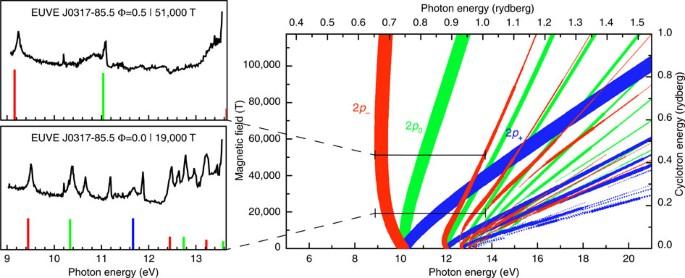Figure 3: Field dependence of hydrogen Lyman series for both Faraday and Voigt geometry. The strongest transitions are labelled according to their upper state. The magnitude of the dipole matrix element and polarization are indicated, respectively, by the thickness and colour of the lines (red, circularσ+for Faraday geometry, that is,k||B; blue, circular σ–for Faraday geometry; green,πztransitions for Voigt geometry that is,k┴B). The spectra are taken from ref.6. The field associated with each spectrum has been chosen for the best fit without regard for the astrophysical models of the temperature and so on, as forFig. 1. Figure 3: Field dependence of hydrogen Lyman series for both Faraday and Voigt geometry. The strongest transitions are labelled according to their upper state. The magnitude of the dipole matrix element and polarization are indicated, respectively, by the thickness and colour of the lines (red, circular σ + for Faraday geometry, that is, k || B ; blue, circular σ – for Faraday geometry; green, π z transitions for Voigt geometry that is, k ┴ B ). The spectra are taken from ref. 6 . The field associated with each spectrum has been chosen for the best fit without regard for the astrophysical models of the temperature and so on, as for Fig. 1 . Full size image The experimental and theoretical results are compared in Fig. 2 and Table 2 . The calculation is in excellent agreement with the donor experiment, in both energy and polarization. There is also a striking correspondence between the calculated donor Lyman series ( Fig. 2 ) and that for hydrogen ( Fig. 3 ), especially between the circularly polarized transitions shown in red and blue. 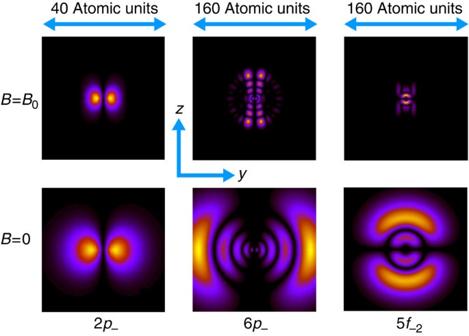Figure 4: Field dependence for some representative wavefunctions. The colour maps showy–zplane cross-sections of probability density for hydrogen wavefunctions. The length scale of the panels is indicated at the top. The extremely strong mixing due to the field is evident from the drastic changes in shape. The equivalent wavefunctions for donors withB||zare almost indistinguishable apart from a shrinkage of thezdimension length scale by a factor √γ~0.5 due to the anisotropy, and the atomic unit of length is now 3.17 nm. The 2p–and 6p–are clearly visible in the donor Lyman spectrum (Fig. 2), while the 5f–2state is forbidden for Lyman transitions. Figure 4 shows the very strong field-induced mixing, evident from the completely different wavefunction shapes at high field. At n =6, the states have a radius of 36 Bohr radii, or 114 nm, which corresponds to the average spacing between the donors (110 nm for the sample used) so that adjacent wavefunctions overlap, leading to broadening of the transitions. These wavefunctions are among the largest in radial extent ever investigated in the solid state, and for a free hydrogen atom to have a similar radius would require n ~45. Table 2 Calculated transition energies compared with experiment. Full size table Figure 4: Field dependence for some representative wavefunctions. The colour maps show y–z plane cross-sections of probability density for hydrogen wavefunctions. The length scale of the panels is indicated at the top. The extremely strong mixing due to the field is evident from the drastic changes in shape. The equivalent wavefunctions for donors with B || z are almost indistinguishable apart from a shrinkage of the z dimension length scale by a factor √ γ ~0.5 due to the anisotropy, and the atomic unit of length is now 3.17 nm. The 2 p – and 6 p – are clearly visible in the donor Lyman spectrum ( Fig. 2 ), while the 5 f –2 state is forbidden for Lyman transitions. Full size image Influence of anisotropic crystal environment in Si:P There are also some notable differences between Figs 2 and 3 . The donors have a number of additional transitions, shown in cyan, that at first sight do not correspond with hydrogen, some transitions that ought to be forbidden for light incident along the field axis (the linearly polarized hydrogen transitions on Fig. 3 , shown in green, such as the 2 p 0 are forbidden for Faraday geometry), and anti-crossings in these transitions. These effects all arise from the fact that while the hydrogen Hamiltonian is spherically symmetric, the donor electron experiences the periodic environment of the cubic crystal host. The constant energy surface in momentum space for electrons in vacuum is a sphere centred at the origin, whereas in silicon there are six equivalent conduction band valleys ( Fig. 2d ) (electrons with zero group-velocity have non-zero phase velocity—an effect of the periodic medium). The valleys are ellipsoidal, that is, anisotropic, and characterized by γ=m t /m l where m t and m l are the transverse and longitudinal effective masses. As a result of the donor anisotropy ( γ ≠1), some degeneracies are lifted at zero field, so that, for example, the 2 p 0 state is unpolarized and at lower energy than the 2 p ± . Anisotropy produces an additional degree of freedom; the angle between the magnetic field and the valley axis. For free hydrogen atoms with spherical symmetry, we are at liberty to choose to quantize the angular momentum along the magnetic field, that is, B =(0,0, B z ). If the silicon sample is mounted with the field in the [001] crystallographic direction then two of the valleys (valleys 1 and 2 in Fig. 2d ) have B || z , where z is the valley axis direction, whereas the other four have B ┴ z . Anisotropy is the origin, for example, of the transition in Fig. 2 that starts at 39.2 meV at zero field but shows no linear Zeeman shift—it is the 2 p ± x for B || x (the subscript x on the level designation indicates the valley orientation). Ground state central cell correction and field dependence The central unit cell of the silicon crystal where the donor atom sits has some strain and rearrangements of the electron cloud that break the host periodicity. These effects are strongly localized and do not extend more than a unit cell. Their net effect is to cause a short-range change in the potential additional to the hydrogenic Coulomb potential, which only affects states with significant amplitude at the centre, that is, donor states that have s -orbital character. In our Lyman series absorption experiment, this quantum defect only affects the ground 1 s state. The observed transition energies ( Fig. 2 ) are all larger than 1 Rydberg, that is, the extra potential is attractive. This observation implies that this wavefunction has a smaller extent than predicted by scaling from hydrogen, which reduces the already small tuning with field (because H 2 =½ A 2 scales with r 2 ). We therefore took the 1 s state to be field independent. We anticipate that the main improvements that can be made to the theory include small adjustments in the parameters, and a better calculation of the ground state and its field dependence, which must include proper treatment of the effects of the central cell correction. Quadratic versus anisotropic linear Zeeman effect Because we have used much higher field and higher quality samples than previous donor spectroscopy [33] , [37] , [38] , we have also resolved new anti-crossings separately induced by either the linear or quadratic Zeeman couplings for the same low quantum number states important in white dwarf spectra ( Fig. 1 ). These anti-crossings are very sensitive tests for the theory, and allow direct experimental measurement of the matrix elements of the Zeeman interaction. For the crystal orientation examined here (that is, [001]), there are examples of anti-crossings that are purely due to the same quadratic Zeeman coupling observed for free hydrogen, while others are purely due to the linear Zeeman coupling introduced by the anisotropy. Looking at the experimental data of Fig. 2 , we can clearly see the anti-crossing of the 2 p ± x line and the 3 p 0 x line at 14 T, with splitting 1 meV. As the dominant basis-state components in the wavefunction are p ± and p 0 , respectively, the term in the Hamiltonian responsible for the anti-crossing clearly couples Δ L =0 and Δ m =±1 (where L is the orbital quantum number), and such terms are not present for hydrogen—it is only produced by the linear Zeeman effect in the presence of anisotropy. Anti-crossings due to this same linear Zeeman coupling may be observed for 2 p ± x and 3 p ± x with 4 p 0 x (with much smaller radial overlap and hence smaller splitting). The downwards shift of 2 p 0 x above 15 T results from similar coupling with 2 p ± x (with large radial overlap). Turning to the quadratic Zeeman Hamiltonian, we observe anti-crossings with Δ m =0 and Δ L =±2 that are entirely due to this coupling, and the same terms are present both in free hydrogen and the silicon donor with B || z . An example is evident in the p – series (red lines on Figs 2 and 3 ), in which transitions gain and lose strength as a function of field. The p – series is coupled by the quadratic Zeeman interaction to the f – (and h – and so on) series, and whereas Lyman transitions from 1 s to p – are dipole allowed, transitions to f – are forbidden. The f – states have the stronger field dependence and the 4 f – cuts through the p – series leaving gaps. 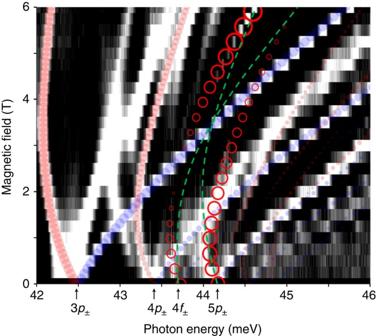Figure 5: Quadratic Zeeman-induced anti-crossing. A detail around 44 meV and 3.5 T of the Si:P absorption (Fig. 2) is shown in white. Superimposed are the theoretical circularly polarized transitions (that is, those which have direct correspondence with free hydrogen): red open/solid symbols, Δm=−1; blue solid symbols, Δm=+1 (and diameter proportional to the magnitude of the dipole matrix element). The excellent agreement between the experiment and theory is evident. The red open symbols highlight the 4f–(starts at 43.7 meV at 0 T) and 5p–(starts at 44.2 meV). The transition 1sto 4f–is only weakly allowed by the anisotropy (it is strictly forbidden atB=0 in hydrogen), while the 5p–is strongly allowed. The transitions anti-cross at about 3.5 T and so that the 4f–line gainsp–character, while the 5p–gainsf–character. The dashed lines are guides to the eye, indicative of the positions of the two levels without their mutual interaction. Figure 5 ( Supplementary Data 3 ) shows a detail of Fig. 2 around the anti-crossing of the 4 f – with the 5 p – . Figure 5: Quadratic Zeeman-induced anti-crossing. A detail around 44 meV and 3.5 T of the Si:P absorption ( Fig. 2 ) is shown in white. Superimposed are the theoretical circularly polarized transitions (that is, those which have direct correspondence with free hydrogen): red open/solid symbols, Δ m =−1; blue solid symbols, Δ m =+1 (and diameter proportional to the magnitude of the dipole matrix element). The excellent agreement between the experiment and theory is evident. The red open symbols highlight the 4 f – (starts at 43.7 meV at 0 T) and 5 p – (starts at 44.2 meV). The transition 1 s to 4 f – is only weakly allowed by the anisotropy (it is strictly forbidden at B =0 in hydrogen), while the 5 p – is strongly allowed. The transitions anti-cross at about 3.5 T and so that the 4 f – line gains p – character, while the 5 p – gains f – character. The dashed lines are guides to the eye, indicative of the positions of the two levels without their mutual interaction. Full size image Having successfully verified the theory of hydrogen in high magnetic fields, we can return to the consideration of the white dwarf star spectra in Fig. 1 . The centre panel shows the calculated hydrogen spectrum at each magnetic field with the dipole strength of each transition reflected in the width of the line. For the six magnetic white dwarfs shown, we have selected the magnetic field that best fits the measured spectrum. There is a good degree of agreement for all spectra and where extra or missing features are present, we can be confident that other effects are responsible (such as, for example, other species or strongly inhomogeneous magnetic fields). In summary, we have experimentally investigated the spectroscopy of a solid-state analogue of hydrogen in conditions equivalent to the surface of the highest field magnetic white dwarf known. The calculated state energies, their anti-crossings, and the selection rules show excellent agreement with experiment up to the highest fields, thus validating the theoretical approach and providing confidence in its use for modelling astrophysical data. The simple scaling between the binding energies for Si:P and hydrogen is extremely well known, and here we show that much more subtle use can be made of it for measurement of Zeeman couplings. These quadratic Zeeman couplings and anti-crossings are responsible for the complexity of the predicted field dependence of the Balmer spectrum ( Fig. 1 ), and although the effect of the quadratic Zeeman interaction has been detected in both free atoms [1] , [15] and solids [28] , [29] , [33] , [34] , [35] , [37] , [38] , its characteristic anti-crossings with Δ m =0 and Δ L =±2 have not been observed previously (and neither have the purely linear Zeeman, B ┴ z anisotropy induced, anti-crossings with Δ m =±1 and Δ L =0). The results show that silicon donors provide an excellent laboratory material for studying effects of atomic physics that have previously been beyond the capability of laboratory equipment and available for study only in extreme astrophysical phenomena. We propose that analogues of helium (such as sulphur or selenium in silicon [36] ) or H 2 (phosphorus pairs), where the theory is yet more difficult, will prove critical to underpinning confident interpretation of other white dwarf spectra. The analogues are also likely to be the only way to study new kinds of magnetic chemical bonds [19] . Our scheme also opens the way to use solid-state systems to investigate quantum effects in a regime where forces manifesting spherical and cylindrical symmetry compete equally. Experimental methods The sample used for Fig. 2a was a 500-μm-thick float zone grown monocrystalline silicon with a phosphorus density of 8 × 10 14 cm −3 , and a residual concentration of other donors and acceptors below 10 13 cm −3 . It was polished to a 1° wedge, and mounted in helium exchange gas at T =2.2 K. Far-infrared radiation from a Fourier transform interferometer (Bruker IFS-113v), was brought to the sample by an evacuated beam line and focusing cone, and the transmission was detected by a liquid-helium-cooled Si-composite bolometer. The unapodized spectral resolution of Fig. 2a was 0.04 meV, confirmed by the residual presence of water vapour absorption lines of this width. The sample exhibits phosphorus donor absorption lines of width 0.09 meV and this is limited by the natural isotopic variation of surrounding silicon atoms (and can be reduced somewhat by purification [29] ). The lifetime broadened line width is 0.008 meV (refs 30 , 31 ). The signal dependence on magnetic flux density B was determined with a 33 T (0.33 MG) water-cooled Bitter magnet, with the field axis, the light propagation direction and the normal to the sample plane all parallel, that is, the Faraday geometry [23] . For polarized experiments, a wire grid polarizer and an x -cut quartz quarter wave plate were mounted with optical axes at 45° to each other directly on top of the sample. The wave plate bandwidth covered only the 2 p 0 and 2 p − transitions. Each transmission interferogram was Fourier transformed, normalized with the median spectrum to remove the water lines, then inverted, and finally offset so that the baseline corresponds to the field applied. No smoothing or other processing has been used. The raw interferogram data for Fig. 2a and Fig. 5 are provided in Supplementary Data 1–3 , respectively. The data consist of interferograms in columns. Each interferogram has been averaged 30 times. The first row of each data matrix refers to the magnetic field value, while the first column indicates the step number, which is in power-of-two multiples of the HeNe laser wavelength that is, 16 × 632.8 nm. A tab is used to separate data within the rows. The length of the interferogram determines the resolution, which is different for each figure/file. The samples (and field resolution) used for each figure are different. All samples are P doped with the growth direction of <100>. All were 500 μm thick and polished to 1° wedge. Further details are on growth method and doping concentration are provided with each Supplementary Data file. Theoretical methods For the theoretical calculations, we used a Lanczos procedure to find the radial wavefunctions exactly [37] . The main alternative approach would have been a variational calculation [38] . The advantage of the latter method is that it does not require large matrix diagonalization. However, the disadvantage is that it requires a very large number of fitting parameters and is therefore not predictive. It has also been shown [37] , [38] that this method does not easily allow separation of linear and quadratic Zeeman terms at high fields. The exact diagonalization method, although it requires large matrices, requires no fitting and it accurately predicts the results for any field direction, it can identify the different contributions to the anti-crossings and it can be used to produce the wavefunctions and matrix elements for the transitions. Because of the mass anisotropy, the zero-field Hamiltonian for silicon is, in scaled atomic units ( Table 1 ), The primed coordinates represent the laboratory frame, and we make a coordinate transformation, [37] so that the kinetic energy operator is isotropic (and consequently the Coulomb potential is now anisotropic): where and θ is the polar zenith angle (that is, angle down from the z axis) in the transformed frame. We write the wavefunction as a series of functions in separated polar coordinates where Y L,m are the spherical harmonics. The U L,m are the wavefunctions to be found. Using the Y L,m as the basis, the Schrödinger Equation using the Hamiltonian of equation 4 in matrix form is where E is the energy and . F L,m,L′,m′ is zero unless m=m ′ and L has the same parity as L ′, so equation 5 produces independent series of levels according to m and parity of L . The values of F L,m,L′,m′ were found by numerically calculating the overlap integral of the spherical harmonic functions, and the secular equation was set up using the finite element approximation to the second derivative. To find the lowest energy-bound states for any given parity and m , this large matrix diagonalization problem was solved using the Lanczos numerical procedure, encoded in ARPACK library routines for Fortran. In silicon donors, we choose z to be along the valley axis, and in general, the field in the laboratory frame, B ′, can now have components in the xy plane. We choose the symmetric gauge [1] , A =½ B × r , and for donors the apparent magnetic field in the transformed frame is [36] The linear Zeeman Hamiltonian is where , L is the angular momentum and are the raising and lowering operators. The quadratic Zeeman Hamiltonian is in which we substituted the Cartesian definitions of the spherical harmonics. The matrix elements of L z lead to an additional diagonal term in equation 5, and is the main contribution to the Zeeman effect at small field along z , and those of Y 0,0 lead to diagonal terms quadratic in field (for all field directions). The matrix elements of L ± , which appear for non-zero B xy , couple states with Δ m =±1, and Δ L =0. The matrix elements of Y 2, m between the basis states are given by Gaunt Coefficients that we evaluated analytically using Wigner 3j symbols. The Y 2,0 term couples states with Δ m =0 and Δ L =0,±2 and appears for all field directions (except to the crystal axis); Y 2,±1 couples states with Δ m =±1 and Δ L =0,±2 and appears when B is neither parallel nor perpendicular to z ; and Y 2,±2 couples states with Δ m =±2 and Δ L =0,±2 and appears when there is a component of field in the xy plane. The Zeeman effect in hydrogen and silicon donors with B || z For free hydrogen atoms, or for B ′ along [001] for silicon donors, we are left only with L z terms in H 1 and Y 0,0 and Y 2,0 terms in H 2 . Of these, only Y 2,0 produces off-diagonal terms. The non-zero off-diagonal matrix elements allow coupling by the magnetic field of spherical harmonic basis states with Δ m =0 and Δ L =0,±2. This is the same set that is coupled by f in the case of donors in silicon, so the donor and hydrogen problems are therefore of the same complexity and can be separated for each different value of m and L parity independently. We solved it using a Lanczos procedure just as for donors in zero field. Using the spherical harmonics up to L =15 as a basis was sufficient for the Lyman series, but L =30 was found to be necessary for the Balmer series. The Lyman calculations of Figs 2 , 3 took a few tens of minutes on a standard laptop. Convergence tests show that the results are accurate to better than 1 part in 10 4 for the highest energy transitions shown. The Zeeman effect in silicon donors with B ′ x,y ≠0 For B ′ xy ≠0, H 1 includes L ± terms and H 2 includes Y 2,±1 and Y 2,±2 terms, which break the Δ m =0 selection rule. This leaves only parity of L as a good quantum number, that is, we now have to include in the basis all spherical harmonics of a given L parity in the basis. This greatly increases the complexity of the problem. We used the Lanczos procedure to solve the coupling due to the L z and Y 2,0 terms only, and treated the remaining terms as a perturbation in the new basis of the new wavefunctions. In doing so we included the 10 states with lowest energy for each L parity and m up to m =±6 and we then diagonalised the Y 2,±1 and Y 2,±2 interactions between these states exactly. Transition rates The electric dipole approximation for the transition rate caused by an oscillating electric field ɛ ′ contains the matrix element (in the laboratory frame) of ɛ ′ . r ′ where the field in the transformed frame is . In terms of the spherical harmonics: This contains a sum of Gaunt coefficients, each related to a different light polarization. Note that these transitions involve states with opposite L parity. The calculation therefore requires calculation of both sets of parity states. In the case of B || z , the m states are not mixed, so for the Lyman series ( Figs 2 , 3 ) we only need −1 <m< 1, for the Balmer series ( Fig. 1 ) we need −2 <m< 2 and so on. Figure 2c shows the experimental verification of the selection rules, that is, the reversal of the field direction reverses the sense of circular polarization needed. How to cite this article: Murdin, B.N. et al . Si:P as a laboratory analogue for hydrogen on high magnetic field white dwarf stars. Nat. Commun. 4:1469 doi: 10.1038/ncomms2466 (2013).